Organophotocatalysed synthesis of 2-piperidinones in one step via [1 + 2 + 3] strategy Six-membered N -containing heterocycles, such as 2-piperidinone derivatives, with diverse substitution patterns are widespread in natural products, drug molecules and serve as key precursors for piperidines. Thus, the development of stereoselective synthesis of multi-substituted 2-piperidinones are attractive. However, existing methods heavily rely on modification of pre-synthesized backbones which require tedious multi-step procedure and suffer from limited substitution patterns. Herein, an organophotocatalysed [1 + 2 + 3] strategy was developed to enable the one-step access to diverse substituted 2-piperidinones from easily available inorganic ammonium salts, alkenes, and unsaturated carbonyl compounds. This mild protocol exhibits exclusive chemoselectivity over two alkenes, tolerating both terminal and internal alkenes with a wide range of functional groups. 2-Piperidinones are important core substructures in many pharmaceuticals and natural products (Fig. 1a ) [1] , [2] , [3] , [4] , [5] , [6] , [7] and serve as key precursors or intermediates for the synthesis of multi-substituted piperidines and medicinally relevant compounds [8] , [9] . In particular, medicinal chemists found that N -containing heterocycles, such as 2-piperidinones and derived piperidines are among the second-most prevalent heterocycles in pharmaceutical core structures [1] , [2] , [10] . Classical methods to access this structural motif heavily rely manipulation of cyclic precursors, such as the hydrogenation of unsaturated δ-lactams [11] , [12] , [13] , [14] , [15] , [16] , [17] and oxidation of piperidines (Fig. 1b ) [18] , [19] . However, the tedious multi-step preinstallation of such backbone structures as well as the strong reductive or oxidative conditions severely hampered the application of these methods. Accordingly, stepwise approaches such as annulations from advanced precursors by reduction-cyclization cascade provided an alternative to access multi-substituted 2-pyridinones [20] , [21] , [22] . Although these strategies are useful, they are limited to specific classes of coupling partners, resulting in specific substituted 2-pyridinones with additional manipulation steps required. To this end, Alper developed a dual catalyzed carbonylation of pyrrolidines by ring expansion to form 6-substituted-2-piperidinones using [Co 2 (CO) 8 /Ru 3 (CO) 12 ] [23] . In 2007, Landais reported a Et 3 B/O 2 mediated multi-component process by involving a tandem radical intermolecular additions-lactamization sequence to access 2-piperidinones [24] . In general, existing methods suffer from limited scope and substitution patterns of 2-piperidinones from advanced synthetic intermediates with poor functional group tolerance. Thus, a streamlined protocol to piperidinones with diverse substitution patterns from easily-available and cheap starting materials is highly desirable yet challenging. Fig. 1: Significance and strategies for the synthesis of 2-piperidinones. a Representative bioactive targets containing 2-piperidinone motifs. b Strategies for the synthesis of 2-piperidinones. c Synthetic strategies enabled by radical cation of alkenes. d Photocatalytic [1 + 2 + 3] strategy to 2-piperidinones from alkenes and ammonium salt (This work). Full size image Over the past decades, visible-light enabled chemical bond-forming processes have become an attractive platform for organic synthesis [25] , [26] , [27] , [28] . Nicewicz reported the seminal work on alkene activation by photo-initiated single electron oxidation to facilitate hydrofunctionalization with inert nucleophiles (Fig. 1c ). However, aliphatic amines are not feasible to undergo such hydrofunctionalization of alkenes due to the low oxidative potentials of starting and resultant amines (Fig. 1c ) [29] , [30] , [31] , [32] , [33] , [34] , [35] , [36] , [37] , [38] , [39] , [40] . Recently, our group developed the direct synthesis of aliphatic primary amines enabled by hydroamination of alkenes from ammonium carbonate [41] , [42] . To date, photocatalytic intermolecular functionalizations of alkenes via the cation radical intermediates of alkenes are limited to hydrofunctionalizations [43] , partially due to the fast hydrogen atom transfer process to quench the stable alkyl radical species (Fig. 1c ). To the best of our knowledge, intermolecular trapping of such radicals by C-C bond formation remains elusive [44] , [45] , [46] , [47] , [48] , [49] , [50] . Thus, we question the feasibility of quenching the carbon-centered radicals by intermolecular C–C bond-forming to substantially expand chemical space of this reaction mode. Herein, we report a metal-free photocatalytic [1 + 2 + 3] strategy for the rapid construction of 2-piperidinones from inorganic ammonium salts and alkenes (Fig. 1d ) [51] , [52] , [53] , [54] , [55] . The use of inorganic salts facilitates the selective C–N bond formation over two different alkenes as well as the radical trap of C-C bond-forming process, providing a rapid access to N -unprotected 2-piperidinones from inorganic ammonium salts. Reaction optimization We commenced our studies with 4-fluoro-β,β-dimethylstyrene 1a and methyl α-phenylacrylate 2a to probe the feasibility of this [1 + 2 + 3] strategy. 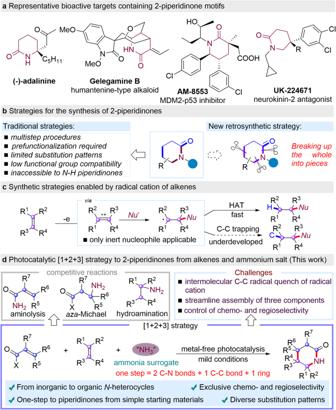Fig. 1: Significance and strategies for the synthesis of 2-piperidinones. aRepresentative bioactive targets containing 2-piperidinone motifs.bStrategies for the synthesis of 2-piperidinones.cSynthetic strategies enabled by radical cation of alkenes.dPhotocatalytic [1 + 2 + 3] strategy to 2-piperidinones from alkenes and ammonium salt (This work). After extensive optimization of reaction parameters, the use of [Mes-3,6- t -Bu 2 -Acr-Ph] + BF 4 − (2.5 mol%) as catalyst, ammonium acetate (3.0 equiv) as nitrogen source and LiBF 4 (1.0 equiv) as additive in CH 3 CN/PhCl (10:1) under blue LED irradiation at room temperature was defined as standard conditions (Table 1 , entry 1), providing the desired 2-piperidinone 3a in 88% yield with a 3.7:1 dr. 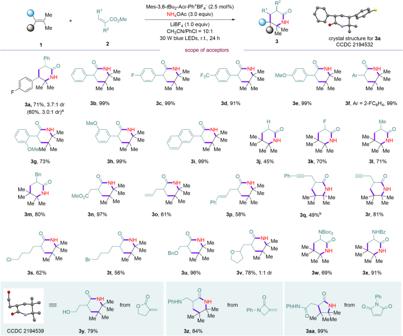Fig. 2: Scope of the acceptors. The reaction was conducted using1(0.1 mmol),2(0.2 mmol) under standard conditions unless otherwise noted. Diastereomeric ratio (dr) was determined by1H NMR of crude mixture of the reaction. Isolated yield after flash chromatography. The disordered part, solvent molecules and hydrogen atoms of crystal structures have been omitted for clarity, for details, see Supplementary Figs.15and16.aCorresponding Weinreb amide was used.b5 mol% photocatalyst was used. The structure and major isomer of 3a were confirmed by X-ray diffraction analysis. The use of ammonia surrogate is essential for this reaction. 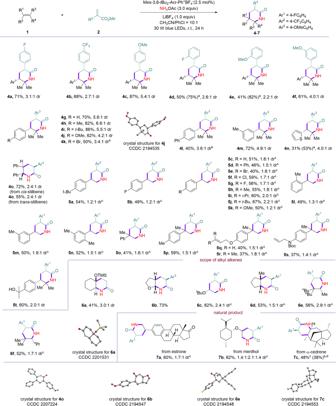Fig. 3: Scope of alkenes. The reaction was conducted using1(0.1 mmol),2(0.2 mmol) under standard conditions unless otherwise noted. Diastereoisomeric ratio (dr) was determined by1H NMR of crude mixture of the reaction. Isolated yield after flash chromatography. The disordered part, solvent molecules and hydrogen atoms of crystal structures have been omitted for clarity. For more details, see Supplementary Figs.17–24.aYield based on the recovery of alkenes.b5 mol% PC was used.cThe reaction was conducted using1(0.1 mmol),2(0.2 mmol), PC (5 mol%), NH4OAc (0.3 mmol), LiBF4(0.1 mmol) in CH3CN:PhCl = 100:1 (10.0 mL CH3CN).dThe reaction was conducted on 2.0 mmol scale. Other ammonium salts could mediate the desired process, albeit leading to the formation of 3a in inferior yields (Table 1 , entries 2–6 and Supplementary Table 3 ). Other acridinum-based photocatalyst proved to be less effective, delivering 3a in 54–61% yields (Table 1 , entries 7–8). Moreover, additive effect showed a significant impact on the diastereoselectivity. In the absence of LiBF 4 , 3a was obtained in comparable yield (80% yield) with only 2.6:1 dr (Table 1 , entry 9). The use of other Lewis acids or Lewis bases as additive provided 3a in lower efficiency and/or diastereomeric ratios (Table 1 , entries 10–14 and Supplementary Table 8 ). Control experiments revealed that both photocatalyst and light irradiation are necessary for the [1 + 2 + 3] transformation (Table 1 , entry 15). Table 1 Condition evaluation of the reaction a Full size table Substrate scope After identifying the optimized reaction conditions, we set to explore the scope of this [1 + 2 + 3] strategy enabled 2-piperidinone synthesis. First, the scope of radical acceptor was tested and the results are summarized in Fig. 2 . Diverse α-aryl acrylate with para - ( 3a – 3e ), ortho - ( 3f and 3g ) and meta - ( 3h ) substituents on the aromatic rings were all well-tolerated, giving the desired 2-piperidinone products in excellent yields (71–99%). In addition, acrylamides could be employed as the acceptor to undergo coupling and cyclization to give 3a in 60% yield. Moreover, fused aryl, alkyl, fluoro-, and benzyl substituted acrylates were all good substrates, affording diverse substitution patterns at 3-position of 2-piperidinones ( 3i–3m ) in good yields. Notably, esters, terminal and internal alkenes, terminal and internal alkynes were tolerated ( 3n – 3r ) under this metal-free conditions. The reaction underwent chemoselective [1 + 2 + 3] reaction to deliver desired products ( 3n – 3r ) in 49–97% yields, leaving chemical space for further elaboration. Halides and ether containing acrylates were successfully involved in the reaction, furnishing corresponding 2-piperidinones ( 3s – 3v ) in 56–96% yields. Amides without or with free protons are both good substrates in the reaction, delivering 3w and 3x in 69% and 91% yields, respectively. Interestingly, vinyl γ-lactone like Tulipalin A could be applied to this reaction, giving 3 y in 79% yield. The structure of 3 y was confirmed by X-ray diffraction analysis. Methylene β-lactam underwent the desired reaction to furnish 3z in 84% yield. Non-polarized electron-deficient alkenes were also compatible under the reaction conditions, delivering corresponding N -phenyl-2-(4,4,5,5-tetramethyl-2-oxopyrrolidin-3-yl)acetamide 3aa in 99% yield. Next, the scope with respect to the other alkenes was examined under the standard conditions. A wide range of functional groups and diverse substitution patterns were amenable in the reaction (Fig. 3 ). Various 2,2-dimethylstyrenes with electron-donating or electron-withdrawing groups reacted smoothly with different alkene acceptors to furnish desired [1 + 2 + 3] products ( 4a – 4n ) in exclusive regioselectivity and good yields with 2.2:1-6.6:1 dr. Notably, both configurations of stilbene were applicable in the reaction, delivering 3,5,6-trisubstituted 2-piperdinone 4o in 72% and 55% yields with identical diastereomeric ratio. Fig. 2: Scope of the acceptors. The reaction was conducted using 1 (0.1 mmol), 2 (0.2 mmol) under standard conditions unless otherwise noted. Diastereomeric ratio (dr) was determined by 1 H NMR of crude mixture of the reaction. Isolated yield after flash chromatography. The disordered part, solvent molecules and hydrogen atoms of crystal structures have been omitted for clarity, for details, see Supplementary Figs. 15 and 16 . a Corresponding Weinreb amide was used. b 5 mol% photocatalyst was used. Full size image Fig. 3: Scope of alkenes. The reaction was conducted using 1 (0.1 mmol), 2 (0.2 mmol) under standard conditions unless otherwise noted. Diastereoisomeric ratio (dr) was determined by 1 H NMR of crude mixture of the reaction. Isolated yield after flash chromatography. The disordered part, solvent molecules and hydrogen atoms of crystal structures have been omitted for clarity. For more details, see Supplementary Figs. 17 – 24 . a Yield based on the recovery of alkenes. b 5 mol% PC was used. c The reaction was conducted using 1 (0.1 mmol), 2 (0.2 mmol), PC (5 mol%), NH 4 OAc (0.3 mmol), LiBF 4 (0.1 mmol) in CH 3 CN:PhCl = 100:1 (10.0 mL CH 3 CN). d The reaction was conducted on 2.0 mmol scale. Full size image 1-Substituted styrenes with diverse substitution patterns on arenes are good substrates in the reaction. Electron-donating and electron-withdrawing groups at para -, meta - and ortho -position of arenes are all tolerated, affording 3,5-disubstituted 2-piperidinones ( 5a – 5n ) in synthetic useful yields. 1,1-Disubstituted styrenes could be applied to the reaction to furnish 3,5,5-trisubstituted 2-piperidiones ( 5o – 5s ) in moderate yields. Moreover, the reaction underwent chemoselective functionalization between multiple alkenes ( 5q – 5s ). Furthermore, free alcohol could also be tolerated in the reaction ( 5t ). Notably, vinyl silyl ether was successfully involved in the reaction to give bicyclic 2-piperidinone 6a in 41% yield. Cyclic and acyclic vinyl ethers are both reactive in the reaction, affording bicyclic piperidinone 6b in 73% yield as single diastereomer and 3,5-disubstituted 2-piperidinone 6c in 62% yield. It deserves mentioning that aliphatic alkenes were applicable in the reaction. Cyclic aliphatic alkene was converted to octahydro-2 H -cyclopenta[ b ]pyridin-2-one ( 6d ) in 53% yield. Acyclic alkyl alkenes reacted to give 3,5,5,6-tetrasubstituted 2- piperidinones ( 6e and 6f ) in 56% and 52% yields. Furthermore, the [1 + 2 + 3] strategy was applied to late-stage functionalization of complex molecules. Alkenes derived from natural products, such as estrone, menthol, and α-cedrene were all compatible with the reaction conditions, successfully affording corresponding natural product-based 2-piperidinones ( 7a – 7c ) in 48%-62% yields. Moreover, the reaction could be scaled up to 2.0 mmol, affording 7c in 38% yield. The major isomers of compounds ( 4j, 4o, 6a, 6b, 6e , and 7c ) were confirmed by X-ray diffraction analysis. Control experiments and mechanistic consideration Next, a series of control experiments were carried out to shed light on the reaction mechanism (Fig. 4 ). First, the reaction of 4-(2-methylprop-1-en-1-yl)-1,1′-biphenyl with methyl 2-(4-methoxyphenyl)acrylate was conducted in the presence of a radical scavenger TEMPO under otherwise identical to standard conditions (Fig. 4a , see more information in Supplementary Information). The desired [1 + 2 + 3] reaction was completely shut down, suggesting the involvement of radical nature in the reaction process. The TEMPO-trapped adduct 8 could be observed by HR-MS analysis. Second, an experiment between 1b and methacrylamide was conducted under standard conditions (Fig. 4b ). However, no desired product 3 l was detected, excluding the possibility of preformation acrylamides during the reaction course. Furthermore, the light on-off experiments of 1b and methyl methacrylate was conducted under standard conditions (Fig. 4c ). The results indicated the reaction undergo a catalytic process instead of a radical chain pathway. In addition, fluorescence-quenching experiments were conducted to further probe the reaction mechanism using 4-fluoro-β,β-dimethylstyrene ( 1a ) and methyl 2-(4-fluorophenyl)acrylate ( 2b ) (Fig. 4d ). Stern-Volmer analysis and time-resolved fluorescence spectroscopy (K sv = 48.07 M −1 , k q = 4.34 × 10 9 M −1 s −1 , see Supplementary Information) indicated that this reaction may proceed through a reductive quenching mechanism of Mes-3,6- t Bu 2 -Acr-Ph + BF 4 − by 4-fluoro-β,β-dimethylstyrene. The quantum yield (Φ) of the reaction using 1b and 2b was determined to be 0.75 (Fig. 4e ), indicating the reaction may undergo a catalytic radical process. Yet, a slow chain propagation mechanism cannot be ruled out at this stage [56] . Fig. 4: Control experiments and mechanistic investigations. a Radical quench experiment. b Control experiment with methacrylamide. c Light on-off experiment. d Stern-Volmer fluorescence-quenching analysis. e Quantum yield. Full size image Based on the experimental results and literature precedence [29] , [30] , [31] , [32] , [33] , [34] , [35] , [36] , [37] , [38] , [39] , [40] , [41] , [42] , [43] , [44] , a plausible reaction mechanism was proposed and depicted in Fig. 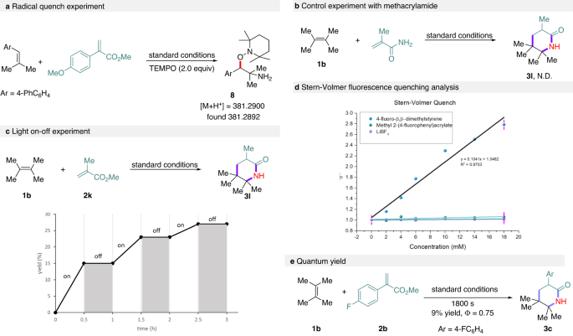Fig. 4: Control experiments and mechanistic investigations. aRadical quench experiment.bControl experiment with methacrylamide.cLight on-off experiment.dStern-Volmer fluorescence-quenching analysis.eQuantum yield. 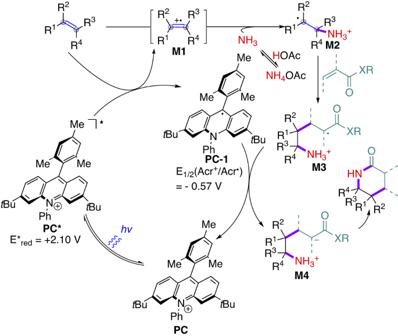Fig. 5: Proposed mechanism. The plausible mechanism for photocatalytic synthesis of 2-piperidinones from alkenes and ammonium salt by [1 + 2 + 3] strategy. 5 . First, excited PC* was generated from PC by visible light irradiation. PC* interacted with the alkenes via single electron oxidation to give radical cation intermediate M1 in conjunction with reduced photocatalyst species PC-1 . M1 is trapped by ammonia released from NH 4 OAc to deliver intermediate M2 . M2 could undergo radical addition with acrylates to generate M3 by C–C bond-formation, which could be further reduced by PC-1 to give intermediate M4 and regenerate PC . Finally, the intramolecular lactamization of M4 generated the desired 2-piperidinone products. Fig. 5: Proposed mechanism. The plausible mechanism for photocatalytic synthesis of 2-piperidinones from alkenes and ammonium salt by [1 + 2 + 3] strategy. Full size image In conclusion, an organophotocatalysed [1 + 2 + 3] strategy for the modular access to unprotected 2-piperidinones has been developed at room temperature. The use of an inorganic ammonium salt as ammonia surrogate enables the construction of N -containing heterocycles from two different alkenes with exclusive chemoselectivity. The reaction forges two C–N bonds and one C–C bond sequentially in one step to construct 2-piperidinones with diverse substitution patterns, providing a streamlined access to 2-piperidinones from easily available starting materials. Mechanistic studies revealed the process was initiated by single electron oxidation of alkenes, followed by an intermolecular nucleophilic attack and intermolecular radical trap to form a C–C bond, representing an intermolecular trap of this carbon radical resulting from radical cation of alkenes to form C–C bonds. We anticipate this reaction will pave the way for this reaction mode to discover new reactions and open the avenue for catalytic transforming inorganic ammonium salts into N -containing organic frameworks. General procedure A for the photocatalytic selective [1 + 2 + 3] construction of 2-piperidinones from alkenes and ammonium salt Under an inert atmosphere, an oven-dried Schlenk-tube equipped with a magnetic stir bar was charged with N -Ph-9-mesityl 3,6-di- tert- butylacridinium tetrafluoroborate (1.4 mg, 2.5 μmol, 2.5 mol%), NH 4 OAc (23.1 mg, 0.3 mmol), LiBF 4 (9.4 mg, 0.1 mmol) and alkene (if solid, 0.1 mmol), CH 3 CN (1.0 mL), alkene (if liquid, 0.1 mmol), acceptor (0.2 mmol) and PhCl (0.1 mL) were added consecutively via syringe. The tube was sealed with a Teflon-coated septum cap, and stirred at ambient temperature under irradiation with 30 W blue LEDs for 12 or 24 h. Upon completion, the reaction mixture was quenched with water and extracted with ethyl acetate. The combined organic phase was concentrated in vacuum. The crude mixture was analyzed by 1 H NMR with PhTMS as internal standard to determine the conversion and was directly purified by column chromatography on silica gel to give the corresponding compound. General procedure B for the photocatalytic selective [1 + 2 + 3] construction of 2-piperidinones from alkenes and ammonium salt Under an inert atmosphere, an oven-dried Schlenk-tube equipped with a magnetic stir bar was charged with N -Ph-9-mesityl 3,6-di- tert- butylacridinium tetrafluoroborate (2.9 mg, 5 μmol, 5 mol%), NH 4 OAc (23.1 mg, 0.3 mmol), LiBF 4 (9.4 mg, 0.1 mmol) and alkene (if solid, 0.1 mmol), CH 3 CN (1.0 mL), alkene (if liquid, 0.1 mmol), acceptor (0.2 mmol) and PhCl (0.1 mL) were added consecutively via syringe. The tube was sealed with a Teflon-coated septum cap, and stirred at ambient temperature under irradiation with 30 W blue LEDs for 24 h. Upon completion, the reaction mixture was quenched with water and extracted with ethyl acetate. The combined organic phase was concentrated in vacuum. The crude mixture was analyzed by 1 H NMR with PhTMS as internal standard to determine the conversion and was directly purified by column chromatography on silica gel to give the corresponding compound. General procedure C for the photocatalytic selective [1 + 2 + 3] construction of 2-piperidinones from alkenes and ammonium salt Under an inert atmosphere, an oven-dried Schlenk-tube equipped with a magnetic stir bar was charged with N -Ph-9-mesityl 3,6-di- tert- butylacridinium tetrafluoroborate (2.9 mg, 5 μmol, 5 mol%), NH 4 OAc (23.1 mg, 0.3 mmol), LiBF 4 (9.4 mg, 0.1 mmol) and alkene (if solid, 0.1 mmol), CH 3 CN (10.0 mL), alkene (if liquid, 0.1 mmol), acceptor (0.2 mmol) and PhCl (0.1 mL) were added consecutively via syringe. The tube was sealed with a Teflon-coated septum cap, and stirred at ambient temperature under irradiation with 30 W blue LEDs for 24 h. Upon completion, the reaction mixture was quenched with water and extracted with ethyl acetate. The combined organic phase was concentrated in vacuum. The crude mixture was analyzed by 1 H NMR with PhTMS as internal standard to determine the conversion and was directly purified by column chromatography on silica gel to give the corresponding compound.